A hierarchically assembled 88-nuclei silver-thiacalix[4]arene nanocluster Thiacalix[4]arenes as a family of promising ligands have been widely used to construct polynuclear metal clusters, but scarcely employed in silver nanoclusters. Herein, an anion-templated Ag 88 nanocluster (SD/Ag88a) built from p -tert-butylthiacalix[4]arene (H 4 TC4A) is reported. Single-crystal X-ray diffraction reveals that C 4 -symmetric SD/Ag88a resembles a metal-organic super calix comprised of eight TC4A 4− as walls and 88 silver atoms as base, which can be deconstructed to eight [CrO 4 @Ag 11 (TC4A)(EtS) 4 (OAc)] secondary building units arranged in an annulus encircling a CrO 4 2− in the center. Local and global anion template effects from chromates are individually manifested in SD/Ag88a. The solution stability and hierarchical assembly mechanism of SD/Ag88a are studied by using electrospray mass spectrometry. The Ag 88 nanocluster represents the highest nuclearity metal cluster capped by TC4A 4− . This work not only exemplify the specific macrocyclic effects of TC4A 4− in the construction of silver nanocluster but also realize the shape heredity of TC4A 4− to overall silver super calix. Due to the esthetic structures and a plethora of promising properties, silver nanoclusters have emerged as a hot topic garnering great interests over the last decade. [1] , [2] , [3] , [4] , [5] , [6] , [7] , [8] , [9] , [10] , [11] , [12] However, their synthetic chemistry is still in the embryo, and trial and error is now the most popular synthetic routine. Regarding their assembly, protecting ligand is one of the most important prerequisites we must consider, and the widely recognized candidates are thiols, alkynes, and phosphines, or their combinations. [13] , [14] , [15] Later, the advancements of anion template strategy [16] , [17] , [18] , [19] and geometric polyhedral principle [20] , [21] , [22] promote the rational design and synthesis of silver nanoclusters to a higher level. Compared with the above-mentioned organic ligands bearing single-coordination site, macrocyclic ligands with multiple preorganized coordination sites are much more desired in the construction of silver nanoclusters because of their reinforcement effect originating from the cooperative coordination of multiple binding groups. These considerations are reminiscent of “third generation” calixarenes–thiacalix[4]arenes, which are macrocyclic tetramers of phenols joined by sulfur atoms [23] and have been recognized as a family of good ligands in the assembly of polynuclear metal clusters and cages. [24] , [25] , [26] , [27] Based on the multiple coordination sites of –OH and –S– groups on them, a series of large metal nanoclusters or nanocages, including Co 16 , Co 24 , Mn 24 , Co 32 , Ni 32 , and Ni 40 , have been reported by Liao and Hong groups. [28] , [29] , [30] , [31] , [32] , [33] However, thiacalix[4]arene-protected silver nanocluster is still rudimentary, and only two closely related p -tert-butylthiacalix[4]arene (H 4 TC4A)-capped reductive Ag 34 and Ag 35 nanoclusters have been reported. [34] , [35] Although the coordination sites of H 4 TC4A favor to support silver nanoclusters, the bulky skeleton of H 4 TC4A also brings a big challenge in growth of single crystals, which is very crucial to understand the structural details of both metal core and metal–ligand interface. Except for the ligand selection, oxoanion template plays another dominant role in constructing silver nanoclusters due to the strong directional effect arising from Ag–O interaction. [36] , [37] , [38] , [39] , [40] , [41] In most cases of anion-templated assembly, oxoanions commonly exert the global effect that means the metal ions aggregate around them in a roughly chaotic fashion without any precedence. As we know, shuttlecock-like {M 4 (TC4A)} (M = Mn, Fe, Co, and Ni) is a very common secondary building unit (SBU) in TC4A 4− -capped metal nanoclusters; [42] however, we do not know what is the SBU if metal is switched to silver in the presence of the anion template. More importantly, we are also unclear that whether the as-formed {(template)@Ag x (TC4A)} SBUs can be further reorganized around the oxoanion template again to form the hierarchical motif. Thus, correlating the SBUs and the final structure of TC4A 4− -capped silver nanocluster is very important for understanding their syntheses and assembly mechanism. Considering the rich advantages of H 4 TC4A in coordination chemistry and the powerful anion template effect in silver nanoclusters, we are extending our researches to combine them together in the synthesis of silver nanoclusters. Herein, we present a C 4 -symmetric silver nanocluster (K 2 [(CrO 4 ) 9 @Ag 88 (TC4A) 8 (EtS) 32 (OAc) 8 ]·8CH 3 CN·4DMF; SD/Ag88a ) with a super calix shape containing the [CrO 4 @Ag 11 (TC4A)(EtS) 4 (OAc)] as SBU. Eight SBUs are further cyclized into an Ag 88 cluster around a central CrO 4 2− . This silver nanocluster is the highest-nuclearity metal cluster capped by TC4A 4− . The structural features including the special ligand effect, local and global anion template effects, as well as the hierarchical assembly in SD/Ag88a will be discussed in detail. Structures of SD/Ag88a and SD/Ag88b Briefly, SD/Ag88a was facilely prepared by the reaction of (EtSAg) n , H 4 TC4A, AgOAc, and K 2 Cr 2 O 7 in the mixed solvent system containing acetonitrile, dichloromethane, and DMF at room temperature (Fig. 1 ). The red prism crystals can be crystallized after 2 weeks and collected together by filtration as bulk samples (~10%). The higher-yield synthesis of SD/Ag88a can be achieved using solvothermal reaction at 65 °C (~40%). The AgOAc in the synthesis of SD/Ag88a is very crucial because we have tried the other eight different silver salts available in our laboratory, including AgBF 4 , CF 3 COOAg, CH 3 SO 3 Ag, CF 3 SO 3 Ag, AgNO 3 , AgSbF 6 , PhCOOAg, and p -TOSAg, but none of them can produce SD/Ag88a . Auxiliary EtS − ligand also shows steric hindrance-related influence on the formation of SD/Ag88a because other larger alkylthiols such as t BuSH or i PrSH cannot produce SD/Ag88a under the same assembly condition. Of note, by mixing AgOAc with AgSbF 6 in this system, we can isolate a similar Ag 88 cluster (K 2 [(CrO 4 ) 9 @Ag 88 (TC4A) 8 (EtS) 32 (OAc) 8 (CH 3 CN)]·8CH 3 CN; SD/Ag88b ), but crystallized in monoclinic P 2 1 /c space group. The detailed structure diagrams for SD/Ag88b are shown in Supplementary Fig. 1 . A series of characterization techniques such as single-crystal X-ray diffraction (SCXRD), powder X-ray diffraction (PXRD), Fourier transform-infrared spectroscopy (FTIR), UV–Vis spectroscopy, thermogravimetric analysis (TGA), dynamic light scattering (DLS), energy-dispersive X-ray spectroscopy (EDS), and transmission electron microscopy (TEM) were used in this system (Supplementary Figs. 7 – 17 ). Fig. 1: Synthetic route for super calix of SD/Ag88a . DCM = dichloromethane, DMF = N , N -dimethylformamide. Color legends for objects: red: H 4 TC4A ligand; green: super calix; pink: silver atom; blue: CrO 4 2− ; yellow: the base of super calix. Full size image X-ray diffraction analyses on single crystals (Supplementary Fig. 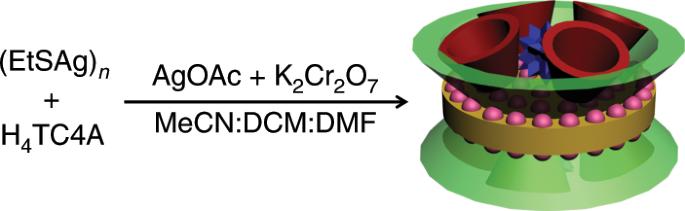Fig. 1: Synthetic route for super calix ofSD/Ag88a. DCM = dichloromethane, DMF =N,N-dimethylformamide. Color legends for objects: red: H4TC4A ligand; green: super calix; pink: silver atom; blue: CrO42−; yellow: the base of super calix. 18 ) of SD/Ag88a and SD/Ag88b revealed that they crystallize in tetragonal P 4/ n and monoclinic P 2 1 /c space groups, respectively (Supplementary Table 1 ). More structural diagrams and crystallographic data plots for them are shown in Supplementary Figs. 19 – 29 . The composition of SD/Ag88a was determined as {K 2 [(CrO 4 ) 9 @Ag 88 (TC4A) 8 (EtS) 32 (OAc) 8 ]·8CH 3 CN·4DMF}. The composition of SD/Ag88b has one more coordinated CH 3 CN on the surface of the cluster compared with SD/Ag88a . The asymmetric unit of SD/Ag88a contains a quarter of Ag 88 cluster and a crystallographic fourfold axis passes through Cr atom of the central CrO 4 2− , whereas no crystallographic symmetry element coincides with the Ag 88 cluster of SD/Ag88b , so a complete molecule was observed in the asymmetric unit. As a result, the overall 88-silver metallic framework of SD/Ag88b is more distorted than that of SD/Ag88a . Due to the structural similarity between SD/Ag88a and SD/Ag88b , we just describe and discuss their structures below by taking SD/Ag88a as a representative. As shown in Fig. 2 , SD/Ag88a looks like a super calix composed of 88 silver atoms, 32 EtS − , 8 TC4A 4− , 8 OAc − , and 9 CrO 4 2− anions. Among them, 88 silver atoms and 8 TC4A 4− ligands roughly constitute the base and wall of the super calix, respectively. The equator diameter and the height of SD/Ag88a are 2.2 and 1.1 nm, respectively, by removing the organic shell. Fig. 2: Single-crystal X-ray structure of SD/Ag88a . a and b Total structures of Ag 88 super calix viewed along two orthogonal directions. The inset in Fig. 2a is the photograph of crystals of SD/Ag88a taken by using a digital camera under the microscope. c and d The skeletal structure of SD/Ag88a by removing all organic ligands and anion templates viewed along two orthogonal directions. Color labels: purple, Ag; yellow, S; gray, C; red, O; green polyhedra, CrO 4 2− . Full size image The metallic skeleton of 88 silver atoms can be divided into eight CrO 4 2− -templated Ag 11 SBUs and each of them is capped by one TC4A 4− with a cone-shaped conformation to form an irregular SBU with a composition of [CrO 4 @Ag 11 (TC4A)(EtS) 4 (OAc)] (Fig. 3a ). The CrO 4 2− plays the local templating effect in such SBU using a μ 10 -κ 3 :κ 3 :κ 2 :κ 2 mode. In the asymmetric unit, there are two Ag 11 SBUs fused together with two TC4A 4− ligands locating in a nearly perpendicular orientation (Supplementary Fig. 2 ). In each cavity of TC4A 4− , one CH 3 CN molecule is encapsulated and its N atom points out of the bigger opening of TC4A 4− (Supplementary Fig. 3 ). The sunken voids formed after removing CH 3 CN molecule from TC4A 4− are clearly shown in Supplementary Fig. 4 . Two crystallographic unique TC4A 4− ligands show different coordination modes using both phenolic hydroxyl and bridging sulfur atoms, μ 6 -κ o 2 :κ o 3 :κ o 3 :κ o 3 :κ s 1 :κ s 1 :κ s 1 :κ s 2 (Fig. 3b ) and μ 7 -κ o 3 :κ o 3 :κ o 3 :κ o 3 :κ s 1 :κ s 1 :κ s 1 :κ s 2 (Fig. 3c ). 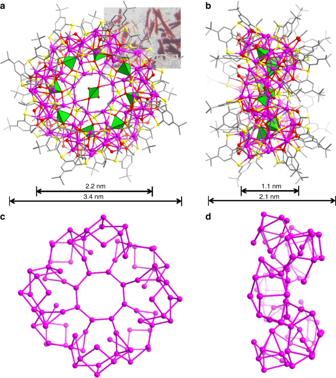Fig. 2: Single-crystal X-ray structure ofSD/Ag88a. aandbTotal structures of Ag88super calix viewed along two orthogonal directions. The inset in Fig. 2a is the photograph of crystals ofSD/Ag88ataken by using a digital camera under the microscope.canddThe skeletal structure ofSD/Ag88aby removing all organic ligands and anion templates viewed along two orthogonal directions. Color labels: purple, Ag; yellow, S; gray, C; red, O; green polyhedra, CrO42−. The Ag–O and Ag–S bond lengths related to TC4A 4− fall in the ranges of 2.255(5)−2.70(1) Å and 2.511(5)−2.753(5) Å, respectively (Supplementary Table 2 ). The OAc − uses bidentate bridging (μ 2 -κ 1 :κ 1 ) mode to coordinate on the Ag 11 SBU (Ag–O: 2.14(2)−2.41(2) Å). Two of four EtS − ligands in each SBU adopt μ 4 mode to cap on Ag 11 SBU (Ag–S: 2.397(5)−2.641(7) Å), whereas the other two (one in μ 3 and another in μ 4 mode) combine with TC4A 4− bridges to consolidate the joints between SBUs (Supplementary Fig. 5 ). One remaining central CrO 4 2− anion (μ 4 -κ 2 :κ 2 :κ 0 :κ 0 ) uses the global templating effect to organize eight Ag 11 SBUs into an annulus finally (Fig. 3d ); thus the best description for SD/Ag88a is {CrO 4 @[CrO 4 @Ag 11 (TC4A)(EtS) 4 (OAc)] 8 }. Although the TC4A 4− ligands effectively cover on SD/Ag88a , we should not neglect the importance of auxiliary small EtS − and OAc − ligands that fill into the coordination unsaturation regions left after TC4A 4− coverage. The argentophilic interactions, featured as the Ag···Ag distances shorter than 3.44 Å falling in the range of 2.825(2)−3.418(2) Å, reinforce the overall Ag 88 skeleton. [43] , [44] , [45] Although linking cationic shuttlecock-like {M 4 (TC4A)} (M = Mn, Fe, Co, and Ni) SBUs by carboxylates can form a very large nanocage with total metal counts more than 30, [29] there are no TC4A 4− -protected metal clusters with nuclearity higher than 80; thus SD/Ag88a is the highest-nuclearity metal cluster capped by TC4A 4− . Compared with the known biggest silver cluster, [Ag 490 S 188 (S t C 5 H 11 ) 114 ], [15] the 88-nuclei silver super calix represents a brand-new structure model in the silver cluster family. Fig. 3: Ag 11 SBU in SD/Ag88a . a The ball-and-stick mode of the structure of [CrO 4 @Ag 11 (TC4A)(EtS) 4 (OAc)] SBU. b , c Two different coordination modes of TC4A 4− ligands. Color labels: purple, Ag; yellow, S; gray, C; red, O; cyan, Cr. d The Ag 88 annulus built from eight Ag 11 SBUs around the central CrO 4 2− anion. Eight Ag 11 SBUs are individually colored. Full size image The packing of SD/Ag88a is also quite interesting and shown in Fig. 4a, c . The Ag 88 super calix is lined in a face-to-face fashion to form a 1D nanotube running along [001] direction. Such packing is mainly dictated by intercluster van der Waals interaction between t -butyl groups on the upper rims and generates some voids as shown in Supplementary Fig. 6 . The distance between adjacent two SD/Ag88a nanoclusters is 23.14 Å based on the separation between two Cr1 atoms. The similar packing was also observed in a chiral lead metal–organic nanotube based on β-cyclodextrin. [46] Interestingly, the packing fashion of SD/Ag88b is completely different from that of SD/Ag88a . The intercluster van der Waals interactions that dominated face-to-side arrangement were found in the packing of SD/Ag88b (Fig. 4b, d ). The centroid separation between two Ag 88 clusters of SD/Ag88b is 26.27 Å. The larger separations between clusters indicated their loose packing that may be sensitive to co-crystallized solvents, although no satisfactory structural model for all solvent positions could be determined from SCXRD analysis. The different weight losses in the first step upon heating in N 2 stream observed in the TGA curves suggested the different solvent-filling in the crystals (Supplementary Fig. 7a ) and the residues after TGA are primarily metallic silver (Supplementary Fig. 7b ). Fig. 4: The packing of SD/Ag88a and SD/Ag88b . Top and side views of the 1D array of SD/Ag88a ( a , c ) and SD/Ag88b ( b , d ). Different Ag 88 clusters are individually colored. The central CrO 4 2− was removed for clarity. Full size image Solution behaviors of SD/Ag88a Mass spectrometry, DLS, and TEM were utilized to check the solution behavior of SD/Ag88a dissolved in CH 2 Cl 2 . The ESI-MS of SD/Ag88a contains five major isotope-distribution envelops ( 1a – 1e ) in the m/z range lower than 4000 (Fig. 5a ). They are trivalent species deduced from the difference (Δ m/z = 0.33) between adjacent isotopic peaks in each envelop. The most dominant envelop centered at m/z = 3038.487 ( 1d ) can be assigned to [(CrO 4 ) 4 @Ag 44 (TC4A) 4 (EtS) 16 (OAc)] 3+ (Calcd. m/z = 3038.513), which is roughly equal to a half of SD/Ag88a but losing one central CrO 4 2− , three OAc − anions, and some guest solvent molecules. In other words, the species 1d is equivalent to four fused Ag 11 SBUs after losing three OAc − anions. Based on the isotope distributions, the envelop 1c centered at m/z = 3009.850 can be assigned to [(CrO 4 ) 4 @Ag 43 (TC4A) 4 (EtS) 14 (OAc) 2 (CH 2 Cl 2 )] 3+ (Calcd. m/z = 3009.859). Interestingly, the m/z spacing between 1a and 1c , 1b and 1d , and 1d and 1e is 55.30 or 55.96, which can be attributed to the mass of one AgOAc divided by the charge state of +3, indicating the coordination–dissociation equilibrium between them involving losing or gaining one AgOAc unit. In the m/z range higher than 4000, we also observed two weak but recognizable peaks centered at 4503.247 ( 1f ) and 4587.207 ( 1g ). After checking the spacing of adjacent isotopic peaks, we found that 1f and 1g are divalent species and can be assigned to [(CrO 4 ) 4 @Ag 43 (TC4A) 4 (EtS) 16 (OAc)] 2+ ( 1f , Calcd. m/z = 4503.318) and [(CrO 4 ) 4 @Ag 44 (TC4A) 4 (EtS) 16 (OAc) 2 ] 2+ ( 1g , Calcd. m/z = 4587.277), respectively. 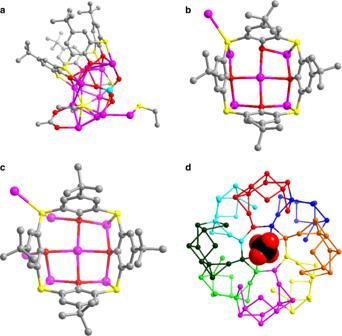Fig. 3: Ag11SBU inSD/Ag88a. aThe ball-and-stick mode of the structure of [CrO4@Ag11(TC4A)(EtS)4(OAc)] SBU.b,cTwo different coordination modes of TC4A4−ligands. Color labels: purple, Ag; yellow, S; gray, C; red, O; cyan, Cr.dThe Ag88annulus built from eight Ag11SBUs around the central CrO42−anion. Eight Ag11SBUs are individually colored. The detailed formulae of 1a – 1g are listed in Supplementary Table 3 . Fig. 5: Positive-ion ESI-MS and proposed solution assembly mechanism of SD/Ag88a . a Positive-ion ESI-MS of SD/Ag88a dissolved in CH 2 Cl 2 . Inset: the expanded experimental and simulated isotope-distribution patterns of 1a – 1g . b The proposed solution assembly mechanism for SD/Ag88a . Full size image To rule out the possible fragmentation pathway of Ag 88 cluster occurred in ESI-MS measurement, we also used DLS and TEM to examine the original CH 2 Cl 2 solution of SD/Ag88a . Both Supplementary Figs. 8 , 9a show some particles with diameters smaller than SD/Ag88a , which clearly suggest that the fragmentation happens in the course of dissolution instead of the ESI-MS process. From the above-combined results, we can conclude that (i) partial SD/Ag88a can keep intact but mainly coexists with a half of it in the CH 2 Cl 2 ; (ii) the coordination–dissociation equilibria involving few ligands and AgOAc exist in this system; (iii) the encapsulation of the central CrO 4 2− may not happen until the final stage enclosing the overall Ag 88 super calix from two halves of Ag 44 fragments. Based on the above structural analysis and the cluster fragmentation path revealed by mass spectrometry, we can retrodict a growth route for SD/Ag88a from bowl-like Ag 11 SBU, a tetrameric semicircular Ag 44 fragment to the final octameric circular Ag 88 super calix (Fig. 5b ). UV–Vis spectra and photocurrent response properties As shown in Fig. 6a , the solid-state UV–Vis spectra of SD/Ag88a , SD/Ag88b, and (EtSAg) n precursor were measured at 250–1000 nm at room temperature. The (EtSAg) n precursor looks yellow to the naked eye, whereas the SD/Ag88a and SD/Ag88b appear to be dark red. Both SD/Ag88a and SD/Ag88b show similar double-hump absorption profile, one narrow peak at ca. 340 nm, and one broad peak starting from ca. 370 to 800 nm. The absorption peak at 340 nm can be attributed to the n → π* transition of EtS − , as similarly observed in the absorption spectrum of the (EtSAg) n precursor. The broad absorption band can be attributed to the charge transfer transition from S 3 p to Ag 5 s orbitals, which thus cause 240 and 190 nm redshifts of the absorption edges for SD/Ag88a and SD/Ag88b , respectively, compared with (EtSAg) n . The bandgaps of SD/Ag88a , SD/Ag88b , and (EtSAg) n precursor were determined as 1.37, 1.48, and 2.19 eV, respectively, according to the Kubelka–Munk function (Supplementary Fig. 10 ), which indicates that the aggregation of silver atoms into the cluster can influence the bandgap structures that include broadening of the absorption edge and narrowing of the bandgap. In addition, both SD/Ag88a and SD/Ag88b are almost emission silent at both room temperature and liquid nitrogen temperature. Fig. 6: The UV–Vis spectra and photocurrent responses of SD/Ag88a and SD/Ag88b . a The normalized UV–Vis spectra of SD/Ag88a , SD/Ag88b , and (EtSAg) n precursor in the solid state. Insets are the digital photographs of SD/Ag88a , SD/Ag88b , and (EtSAg) n taken under the ambient environment. b Compared photocurrent responses of blank, (EtSAg) n , SD/Ag88a , and SD/Ag88b ITO electrodes in a 0.2 M Na 2 SO 4 aqueous solution under repetitive irradiation. Full size image Considering the wide visible light absorption, we performed photocurrent measurements for (EtSAg) n , SD/Ag88a , and SD/Ag88b in a typical three-electrode system by coating them on indium-doped SnO 2 (ITO) as working electrodes (platinum wire as the assisting electrode and Ag/AgCl as the reference electrode) and keeping the bias voltage at 0.6 V. The photocurrent experiments were carried out in a 0.2 M Na 2 SO 4 aqueous solution under illumination upon on/off cycling irradiation with LED light (λ = 420 nm; 50 W; intervals of 10 s). Upon irradiation, photocurrent density increases at 0.16, 0.12, and 0.20 μA cm −2 for (EtSAg) n , SD/Ag88a , and SD/Ag88b , respectively (Fig. 6b ), which indicates that the SD/Ag88b possesses the best efficiency in the generation and separation of photoinduced electron/hole pairs in ITO electrodes. [47] The photocurrent density can be still kept after ten on/off cycles, suggesting the response reproducibility. The generation of photocurrent may involve photoinduced charge migration from S 3 p to the Ag 5 s orbits. The stability of the electrode was further proved by the compared IR spectra and PXRD patterns. [48] After the photocurrent tests, both IR spectra (Supplementary Figs. 11 , 12 ) and PXRD patterns (Supplementary Figs. 13 , 14 ) of samples were basically identical to those of original samples, which indicates that these samples did not undergo decomposition in the process of electrode preparation and during the photocurrent measurements. In summary, we have assembled and characterized a silver-organic super calix comprising 88 silver atoms and 8 TC4A 4− ligands. SD/Ag88a is the highest-nuclearity metal cluster based on TC4A 4− . Structural analysis revealed important chromate-templated Ag 11 SBUs, which are further fused into a super calix of SD/Ag88a with a remaining CrO 4 2− sitting on the center. Both local and global anion-templating effects from chromates are clearly manifested in the hierarchical structure of SD/Ag88a . The hierarchical assembly mechanism from bowl-like Ag 11 SBU, a semicircular Ag 44 fragment to the final circular Ag 88 super calix was also revealed by using electrospray mass spectrometry (ESI-MS). The successful installation of TC4A 4− ligand on silver nanocluster exemplifies its powerful chelating ability and macrocyclic effects, which surely open a bright road to assembly of silver nanoclusters using such kind of macrocyclic ligands. Synthesis of SD/Ag88a Method A: the mixture of (EtSAg) n (0.05 mmol, 8.5 mg), H 4 TC4A (0.015 mmol, 10.8 mg), and K 2 Cr 2 O 7 (0.025 mmol, 7.3 mg) were dissolved in mixed solvent of acetonitrile, dichloromethane, and N , N’ -dimethylformamide (6.5 mL, v:v:v = 10:2:1). The mixed solution was stirred for 1 h at room temperature, then AgOAc (0.1 mmol, 16.7 mg) was added to the above mixture for another 3 h of stirring. The red solution was filtrated and evaporated in the dark for 2 weeks. The red prism crystals of SD/Ag88a were obtained in a yield of 10%. 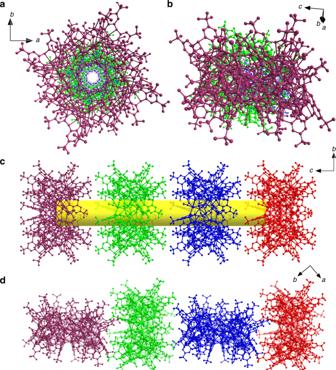Fig. 4: The packing ofSD/Ag88aandSD/Ag88b. Top and side views of the 1D array ofSD/Ag88a(a,c) andSD/Ag88b(b,d). Different Ag88clusters are individually colored. The central CrO42−was removed for clarity. Synthesis of SD/Ag88a Method B: the mixture of (EtSAg) n (0.05 mmol, 8.5 mg), H 4 TC4A (0.015 mmol, 10.8 mg), and K 2 Cr 2 O 7 (0.025 mmol, 7.3 mg) were dissolved in mixed solvent of acetonitrile, dichloromethane, and N , N’ -dimethylformamide (6.5 mL, v:v:v = 10:2:1). The mixed solution was stirred for 1 h at room temperature. To this solution AgOAc (0.1 mmol, 16.7 mg) was added. The reaction continued for further 3 h of stirring, then the red mixture was sealed in a 25-mL Teflon-lined reaction vessel and kept at 65 °C for 2000 min. After cooling to room temperature, the red solution was filtrated and evaporated in the dark for 1 week. The red prism crystals of SD/Ag88a were isolated in a yield of 40%. Elemental analyses calc. 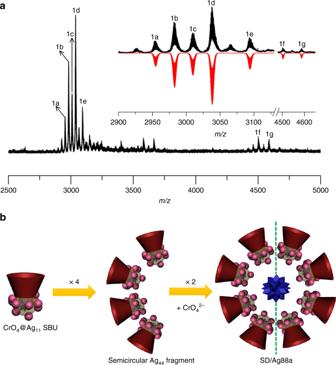Fig. 5: Positive-ion ESI-MS and proposed solution assembly mechanism ofSD/Ag88a. aPositive-ion ESI-MS ofSD/Ag88adissolved in CH2Cl2. Inset: the expanded experimental and simulated isotope-distribution patterns of1a–1g.bThe proposed solution assembly mechanism forSD/Ag88a. 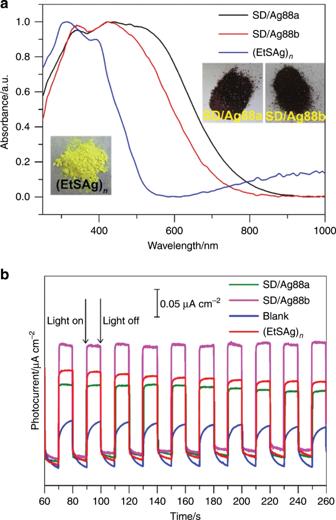Fig. 6: The UV–Vis spectra and photocurrent responses ofSD/Ag88aandSD/Ag88b. aThe normalized UV–Vis spectra ofSD/Ag88a,SD/Ag88b, and (EtSAg)nprecursor in the solid state. Insets are the digital photographs ofSD/Ag88a,SD/Ag88b, and (EtSAg)ntaken under the ambient environment.bCompared photocurrent responses of blank, (EtSAg)n,SD/Ag88a, andSD/Ag88bITO electrodes in a 0.2 M Na2SO4aqueous solution under repetitive irradiation. (found) for SD/Ag88a (C 428 H 588 Ag 88 Cr 9 K 2 N 12 O 88 S 64 ): C, 26.50 (26.51); H, 3.06 (3.08); N 0.87 (0.85)%. Selected IR peaks (cm −1 ): 3382 (w), 2949 (w), 1658 (w), 1550 (w), 1434 (s), 1301 (w), 1245 (m), 1209 (w), 848 (m), 828 (s), 760 (m), 724 (m), 650 (w), 612 (w), 540 (w), 520 (w). Synthesis of SD/Ag88b The synthesis conditions were similar to those described for Method B above, but using AgOAc (0.1 mmol, 16.7 mg) and AgSbF 6 (0.05 mmol, 17.2 mg) instead. Red prism crystals of SD/Ag88b were isolated in a yield of 37%. Elemental analyses calc. (found) for SD/Ag88b (C 418 H 563 Ag 88 Cr 9 K 2 N 9 O 84 S 64 ): C, 26.22 (26.14); H, 2.96 (3.00); N 0.66 (0.59)%. Selected IR peaks (cm −1 ): 2949 (w), 1549 (w), 1472 (w), 1433 (s), 1356 (m), 1304 (m), 1239 (m), 1051 (w), 966 (w), 855 (m), 830 (s), 764 (m), 720 (m), 648 (w), 528 (w).